LRP5/6 directly bind to Frizzled and prevent Frizzled-regulated tumour metastasis How Wnt signalling including canonical and non-canonical pathways are initiated at the cell surface is not completely understood. Here we report that Wnt receptor Frizzled (Frz) and theco-receptors LRP5 and LRP6 (LRP5/6) directly interact with each other and this interaction is regulated by the LRP6 ectodomain. Importantly, through direct binding to Frz, LRP5/6 are able to prevent Frz-regulated non-canonical pathway activation and further non-canonical pathway-mediated tumour metastasis. Knockdown of endogenous LRP5/6 promotes otherwise-nonaggressive tumour cells to migrate in vitro , whereas a soluble recombinant protein of LRP6 ectodomain suppresses migration and metastasis of otherwise-aggressive tumour cells in vitro and in vivo . Furthermore, the expression level of membrane LRP5/6 correlates inversely with metastasis in mouse and human breast cancer. Our study suggests a previously unrecognized mode of receptor interaction, revealing the mechanism of LRP5/6 in inhibition of non-canonical pathway, and a possible clinical use of the LRP6 ectodomain to impede metastasis. Wnt signalling including β-catenin-dependent canonical and β-catenin-independent non-canonical pathways controls animal development and homeostasis, while deregulation of Wnt signalling causes various diseases in humans including cancer [1] , [2] . Wnt–Frz interaction activates the non-canonical pathway, but to activate the canonical pathway, Wnt co-receptors LRP5/6 are also required. The canonical Wnt1 gene was originally identified as a preferential integration site for the mouse mammary tumour virus in virally induced breast tumours [3] . Thereafter, LRP5/6 have been identified to be key for Wnt1-dependent tumour development in the Wnt1 transgenic mouse model [4] , [5] , [6] and LRP6 is often overexpressed in human breast tumours [7] . Thus, the components of the canonical pathway including LRP5/6 are commonly thought to be involved in cancer development as oncogenes. The ectodomain of LRP5/6 is composed of four β-propeller/epidermal growth factor (EGF) repeats (E1-4) and three LDL repeats (LDLR). E1-4 but not LDLR is the binding domain of canonical Wnt ligands and the canonical pathway inhibitor Dkk1 (refs 8 , 9 , 10 , 11 ). So far, the LDLR-binding proteins remain unexplored. The current view is that the close proximity of LRP5/6 and Frz coupled by canonical Wnt ligand binding to E1-4 of LRP5/6 and amino-terminal cysteine-rich domain (CRD) of Frz is needed for canonical pathway activation [2] , [9] . In contrast, Dkk1 promotes the internalization of LRP5/6 via binding with Dkk1 receptor Kremen, making LRP5/6 unavailable for Wnt reception and inhibiting the canonical pathway [12] . In contrast, components of non-canonical pathways including planar cell polarity (PCP) and Wnt/Ca 2+ pathways have been implicated in directly promoting the invasiveness of diverse forms of cancer [13] , [14] , [15] . The non-canonical Wnt5a can promote normal cell motility as well as tumour metastasis through the activation PCP/JNK or Ca 2+ /PKC signalling cascade [16] , [17] , [18] . Thus, non-canonical pathways are involved in cancer development through promoting tumour cell motility. Surprisingly, our present study shows that LRP5/6 are able to prevent Frz-regulated non-canonical pathway activation and thereby non-canonical pathway-mediated tumour metastasis through direct binding to Frz. Our results thus reveal LRP5/6 as a novel metastasis suppressor. LRP6 interacts with Frz independently of Wnt ligands The close proximity of LRP5/6 and Frz coupled by Wnt ligands is currently thought to be required for canonical signal transduction. Clearly, it is difficult for Wnt ligands to simultaneously capture LRP5/6 and Frz if they are far away from each other. We hypothesize that LRP5/6 and Frz are in the same complex at cell surface. Immunoprecipitation (IP)/western blot (WB) analysis revealed that full-length LRP6 interacted with Frz8, and this interaction was not affected by sequestration of Wnt ligands with co-transfected soluble form of Frz8-CRD ( Fig. 1b ). Of note, the transfected Frz8-CRD was sufficient to bind to and interfere with all endogenous Wnt ligands ( Supplementary Fig. 1a ). In contrast, full-length LRP6 did not bind to Frz8-CRD that bound to Wnt3a as previously reported [19] ( Fig. 1c ), and Frz8 did not interact with an unrelated single-span receptor Notch ( Fig. 1d ). These results suggest that LRP6 and Frz8 specifically interact with each other, and this LRP6-Frz8 interaction is Wnt-independent but regulated by regions of Frz8 beyond Frz8-CRD. 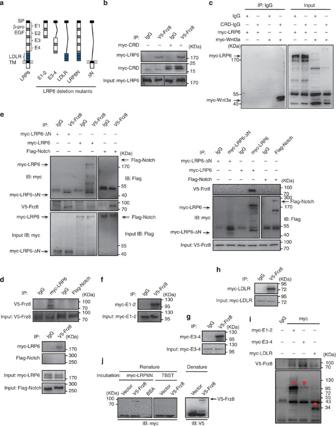Figure 1: LRP6 and Frz8 interact with each other independently of Wnt ligand. (a) Schematic diagram of LRP6 deletion mutants. (b–i) HEK293 cells were transfected with indicated plasmids and harvested for IP/WB analysis after 48 h. IP/WB analysis showed that V5-Frz8 interacted with myc-LRP6, which was not affected by the presence of myc-Frz8-CRD (myc-CRD) (b). myc-LRP6 did not bind to IgG-Frz8-CRD that bound to myc-Wnt3a (c). V5-Frz8 bound to myc-LRP6 (d,e) but not to Flag-Notch (d,e) or myc-LRP6-ΔN (e). IP/WB analysis also showed the interaction of V5-Frz8 with myc-E1-2 (f), myc-E3-4 (g) or myc-LDLR (h), and the interaction of myc-E1-2, myc-E3-4 or myc-LDLR with V5-Frz8 (i). (j) FAR-WB analysis showed the direct interaction of purified myc-LRP6N with V5-Frz8. Figure 1: LRP6 and Frz8 interact with each other independently of Wnt ligand. ( a ) Schematic diagram of LRP6 deletion mutants. ( b – i ) HEK293 cells were transfected with indicated plasmids and harvested for IP/WB analysis after 48 h. IP/WB analysis showed that V5-Frz8 interacted with myc-LRP6, which was not affected by the presence of myc-Frz8-CRD (myc-CRD) ( b ). myc-LRP6 did not bind to IgG-Frz8-CRD that bound to myc-Wnt3a ( c ). V5-Frz8 bound to myc-LRP6 ( d , e ) but not to Flag-Notch ( d , e ) or myc-LRP6-ΔN ( e ). IP/WB analysis also showed the interaction of V5-Frz8 with myc-E1-2 ( f ), myc-E3-4 ( g ) or myc-LDLR ( h ), and the interaction of myc-E1-2, myc-E3-4 or myc-LDLR with V5-Frz8 ( i ). ( j ) FAR-WB analysis showed the direct interaction of purified myc-LRP6N with V5-Frz8. Full size image IP/WB analysis also revealed that LRP6 bound to Frz3 and Frz4 ( Supplementary Fig. 2 ), indicating that LRP6 could potentially interact with various Frz receptors. LRP6 ectodomain interacts with Frz8 To map the regions of LRP6 interaction with Frz8, we generated the truncated mutants of LRP6 including E1-2, E3-4, LDLR and C-terminal of LRP6 (ΔN). IP/WB analysis revealed that Frz8 interacted with full-length LRP6, but not with ΔN or Notch as a negative control ( Fig. 1e ). These results indicate that LRP6 ectodomain but not cytoplasmic domain interacts with Frz8. Moreover, Frz8 interacted with all three ectodomains including E1-2, E3-4 and LDLR ( Fig. 1f–i ). It is known that LRP6 ectodomain E1-2 and E3-4 but not LDLR is able to bind Wnt ligands [8] , [9] , [10] , [11] . Hence, our conclusion that the LDLR domain interacts with Frz8 further suggests that the LRP6–Frz8 interaction is Wnt-independent. To exclude non-specific interaction such as aggregation induced by overexpression, we used FAR-WB analysis that was derived from the standard WB method to detect protein–protein interactions in vitro [20] . As Frz8 protein could not be purified, V5-tagged Frz8 as a ‘prey’ protein was separated by gel electrophoresis and then transferred to a PVDF membrane. The membrane was incubated with a purified soluble form of myc-tagged LRP6 ectodomain (LRP6N) as a ‘bait’ protein, and the FAR-WB analysis showed the direct interaction between LRP6N and Frz8 ( Fig. 1j ). LRP6 ectodomain interacts with Frz8 in living cells We also observed the interaction between LRP6 and Frz8 in living cells using a BRET technique, which is an assay that indicates that the energy donor and acceptor are in close proximity (typically within 100 Å from one another) [21] . Co-transfection of Rluc8-tagged LRP6 (LRP6-Rluc8) with increasing amount of GFP2-tagged Frz8 (Frz8-GFP2) induced an increase in the BRET signals, reaching a plateau at saturating BRET levels ( ∼ 0.06) ( Fig. 2b , black line), which was inhibited by co-transfection with untagged Frz8 or full-length LRP6 in a dose-dependent manner ( Fig. 2c,d ). These results suggest that LRP6 specifically interacts with Frz8. In contrast, co-transfection of LRP6-ΔN-Rluc8 with increasing amount of Frz8-GFP2 led to marginal BRET signals that increased linearly with increasing amount of the receptor-GFP2 added ( Fig. 2b , red line), indicating that the BRET signal between LRP6-ΔN-Rluc8 and Frz8-GFP2 originates from random collisions, and, therefore, the interaction between LRP6 and Frz8 is regulated by LRP6 ectodomain but not its cytoplasmic domain. The BRET activity produced by LRP6-Rluc8 and Frz8-GFP2 was also inhibited by co-transfection with untagged LRP6-ΔC but not LRP6-ΔN in a dose-dependent manner ( Fig. 2e,f ), further suggesting the interaction between LRP6 and Frz8 is regulated by LRP6 ectodomain but not its cytoplasmic domain. Moreover, the BRET activity produced by LRP6-Rluc8 and Frz8-GFP2 was not altered following Wnt3a stimulation ( Fig. 2g ). Co-transfection of LRP6-Rluc8 with an increasing amount of Frz8-ΔN-GFP2 that does not interact with Wnt ligands also resulted in an increase in the BRET ratio ( Fig. 2h ). These results suggest that this LRP6–Frz8 interaction is Wnt ligand-independent but regulated by regions of Frz8 beyond Frz8-CRD. Taken together, these results indicate that this LRP6–Frz8 interaction in living cells is also Wnt-independent but regulated by LRP6 ectodomain and regions of Frz8 beyond Frz8-CRD. 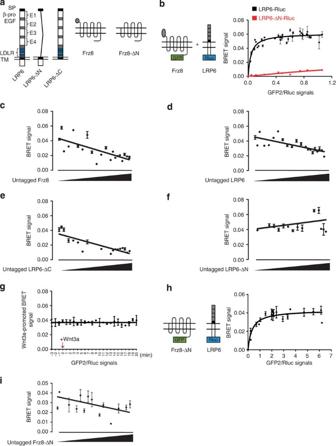Figure 2: LRP6 and Frz8 interact with each other in living cells. (a) Schematic diagram of LRP6 and Frz8 deletion mutants. (b–i) Interaction between LRP6 and Frz8 as assessed by BRET saturation curves and competition assays. In saturation assays, HEK293 cells were co-transfected with a constant DNA concentration of LRP6-Rluc8 (b, black line andh) or LRP6-ΔN-Rluc8 (b, red line) and increasing DNA concentration of Frz8-GFP2 (b) or Frz8-ΔN-GFP2 (h). In competition assays, constant plasmids of LRP6-Rluc8 with Frz8-GFP2 or Frz8-ΔN-GFP2 were co-expressed with an increasing amount of untagged Frz8 (c), Frz8-ΔN (i), full-length LRP6 (d), LRP6-ΔC (e) or LRP6-ΔN plasmid (f). The BRET, total luminescence and total fluorescence were measured 48 h after transfections. The BRET levels are plotted as a function of the ratio of [receptor-GFP2]/[receptor-Rluc8] used as an index for the concentration of receptor-GFP2 constructs expressed. The results are expressed as the mean±s.d. of at least three independent experiments carried out in triplicates. The curves were fitted using a non-linear regression equation assuming a single binding site (GraphPad Prism). Of note, the BRET activity induced by a constant amount of LRP6-Rluc8 and Frz8-GFP2 was not affected by stimulation with Wnt3a (g), and co-transfection of LRP6-Rluc8 with Frz8-ΔN-GFP2 also increased the BRET ratio (h), which was inhibited by untagged Frz8-ΔN (i). Figure 2: LRP6 and Frz8 interact with each other in living cells. ( a ) Schematic diagram of LRP6 and Frz8 deletion mutants. ( b – i ) Interaction between LRP6 and Frz8 as assessed by BRET saturation curves and competition assays. In saturation assays, HEK293 cells were co-transfected with a constant DNA concentration of LRP6-Rluc8 ( b , black line and h ) or LRP6-ΔN-Rluc8 ( b , red line) and increasing DNA concentration of Frz8-GFP2 ( b ) or Frz8-ΔN-GFP2 ( h ). In competition assays, constant plasmids of LRP6-Rluc8 with Frz8-GFP2 or Frz8-ΔN-GFP2 were co-expressed with an increasing amount of untagged Frz8 ( c ), Frz8-ΔN ( i ), full-length LRP6 ( d ), LRP6-ΔC ( e ) or LRP6-ΔN plasmid ( f ). The BRET, total luminescence and total fluorescence were measured 48 h after transfections. The BRET levels are plotted as a function of the ratio of [receptor-GFP2]/[receptor-Rluc8] used as an index for the concentration of receptor-GFP2 constructs expressed. The results are expressed as the mean±s.d. of at least three independent experiments carried out in triplicates. The curves were fitted using a non-linear regression equation assuming a single binding site (GraphPad Prism). Of note, the BRET activity induced by a constant amount of LRP6-Rluc8 and Frz8-GFP2 was not affected by stimulation with Wnt3a ( g ), and co-transfection of LRP6-Rluc8 with Frz8-ΔN-GFP2 also increased the BRET ratio ( h ), which was inhibited by untagged Frz8-ΔN ( i ). Full size image Frz8 inhibits LRP6 function by the Frz8–LRP6 interaction We then examined the effect of Frz8–LRP6 interaction on canonical signal transduction using β-catenin-responsive TOPFLASH reporter gene assay. Co-expression of full-length Frz8 or Frz8-ΔCRD attenuated TOPFLASH activity induced by constitutively active mutant β-catenin-ΔN, indicating an indirect effect of Frz8, which is likely regulated by cross-talk between canonical and non-canonical pathways. However, co-expression of Frz8-ΔC mutant without carboxyl-terminal of Frz8, which has an attenuated capacity to transduce signal to exclude Frz-induced secondary effect, did not affect TOPFLASH activity induced by β-catenin-ΔN ( Fig. 3b ). Thus, we used Frz8-ΔC to examine the effect of Frz8 on LRP6-mediated canonical pathway activation. Co-expression of Frz8-ΔC attenuated TOPFLASH activity induced by full-length LRP6 but not LRP6-ΔN without ectodomain ( Fig. 3c,d ). Because Frz8 binds to full-length LRP6 but not to LRP6-ΔN, the Frz8 inhibition on full-length LRP6-induced TOPFLASH activation is probably through direct binding to LRP6 ectodomain. Indeed, co-expression of Frz8-ΔC also attenuated TOPFLASH activity induced by LRP6 ectodomain-truncated mutant LRP6-ΔE3-4LDLR (including ectodomain E1-2), LRP6-ΔE1-2LDLR (including ectodomain E3-4) or LRP6-ΔE1-4 (including ectodomain LDLR) ( Fig. 3e–g ). Collectively, these results indicate that the inhibitory effect of Frz8 is through direct binding to LRP6 ectodomains. 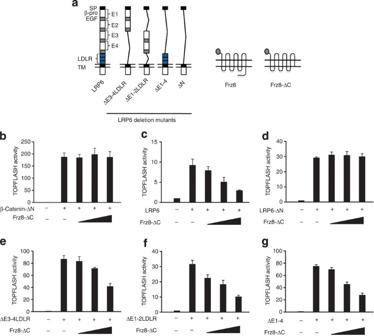Figure 3: Frz8 inhibits LRP6-induced canonical pathway activation by the direct Frz8–LRP6 interaction. (a) Schematic diagram of LRP6 and Frz8 deletion mutants. (b–g) TOPFLASH reporter gene assay. Deletion of the C-terminal domain of Frz8 (Frz8-ΔC) attenuated TOPFLASH activity induced by full-length LRP6 (c), LRP6-ΔE3-4LDLR (e), LRP6-ΔE1-2LDLR (f) or LRP6-ΔE1-4 (g), but not constitutively active mutant β-catenin-ΔN (b) or LRP6-ΔN (d). Values represent mean±s.d. of three experiments. Figure 3: Frz8 inhibits LRP6-induced canonical pathway activation by the direct Frz8–LRP6 interaction. ( a ) Schematic diagram of LRP6 and Frz8 deletion mutants. ( b – g ) TOPFLASH reporter gene assay. Deletion of the C-terminal domain of Frz8 (Frz8-ΔC) attenuated TOPFLASH activity induced by full-length LRP6 ( c ), LRP6-ΔE3-4LDLR ( e ), LRP6-ΔE1-2LDLR ( f ) or LRP6-ΔE1-4 ( g ), but not constitutively active mutant β-catenin-ΔN ( b ) or LRP6-ΔN ( d ). Values represent mean±s.d. of three experiments. Full size image LRP6 ectodomain inhibits Frz8 function We further examined the functional effect of LRP5/6–Frz interaction on Frz-regulated non-canonical signal transduction using stable human liver tumour HepG2 cell line expressing Frz8 (HepG2/Frz8). Stable expression of Frz8 in HepG2 cells activated the non-canonical pathway, resulting in an increase in phospho-c-jun levels and promoting cell migration as shown in matrigel assay, which were attenuated by pretreatment with a soluble recombinant protein of LRP6 ectodomain (LRP6N) (binding to Frz) and Frz8-CRD (sequestration of endogenous Wnt ligands), and a JNK inhibitor ( Fig. 4a–c ). These results suggest the possibility that LRP6 ectodomain prevents tumour cell motility through inhibiting Frz-mediated non-canonical pathway activation. 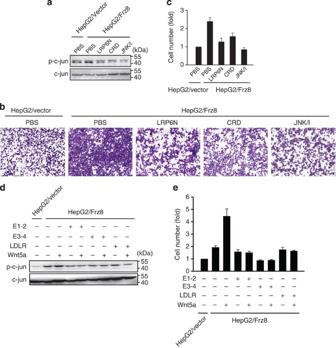Figure 4: LRP6 ectodomain inhibits Frz8-regulated non-canonical pathway activation. (a,d) WB analysis of phospho-c-jun (p-c-jun). Stable expression of Frz8 in HepG2 cells (HepG2/Frz8) increased the level of p-c-jun, which was attenuated by LRP6N (1 μg ml−1), Frz8-CRD-IgG/Fc (CRD) (1 μg ml−1), JNK inhibitor (JNK/I) SP600125 (10 μM) (a) or CM containing E1-2, E3-4 or LDLR (d). Wnt5a further enhanced the level of p-c-jun, which was attenuated by CM containing E1-2, E3-4 or LDLR (d);n=3. (b,c,e) Photoimages of transwell analysis showed increased migrating cells in HepG2/Frz8 cells after 24 h, which was inhibited by LRP6N, CRD or JNK/I (b), or CM containing E1-2, E3-4 or LDLR pretreatment in the upper chamber for 2 h. Cell numbers were counted (c,e). Scale bar, 300 μm. Values represent mean±s.d. of three experiments. Figure 4: LRP6 ectodomain inhibits Frz8-regulated non-canonical pathway activation. ( a , d ) WB analysis of phospho-c-jun (p-c-jun). Stable expression of Frz8 in HepG2 cells (HepG2/Frz8) increased the level of p-c-jun, which was attenuated by LRP6N (1 μg ml −1 ), Frz8-CRD-IgG/Fc (CRD) (1 μg ml −1 ), JNK inhibitor (JNK/I) SP600125 (10 μM) ( a ) or CM containing E1-2, E3-4 or LDLR ( d ). Wnt5a further enhanced the level of p-c-jun, which was attenuated by CM containing E1-2, E3-4 or LDLR ( d ); n =3. ( b , c , e ) Photoimages of transwell analysis showed increased migrating cells in HepG2/Frz8 cells after 24 h, which was inhibited by LRP6N, CRD or JNK/I ( b ), or CM containing E1-2, E3-4 or LDLR pretreatment in the upper chamber for 2 h. Cell numbers were counted ( c , e ). Scale bar, 300 μm. Values represent mean±s.d. of three experiments. Full size image As it is well established that LRP5/6 mutant lacking the cytoplasmic tail is a dominant-negative mutant for canonical Wnt/β-catenin signalling through binding to and neutralizing Wnt ligands [19] , [22] , [23] , [24] , we cannot exclude a possibility that the inhibitory effect of LRP6N on the Frz8-mediated non-canonical pathway activation is via binding to and sequestration of endogenous Wnt ligands. Non-canonical Wnt ligand Wnt5a has been reported not to interact with LRP6 (refs 25 , 26 ), although it has also been reported to be able to interact with LRP5 and Frz4 to activate canonical signalling when LRP5 and Frz4 are overexpressed [25] . Therefore, if LRP6N can also inhibit Wnt5a-induced non-canonical pathway activation, this inhibitory effect should be through the direct binding of LRP6N to Frz. Wnt5a treatment resulted in an increase in phospho-c-jun levels and promoted cell migration in the HepG2/Frz8 cells ( Fig. 4d,e ). All three conditioned media (CM) including E1-2, E3-4 and LDLR impeded the increase in phospho-c-jun levels and cell migration ( Fig. 4d,e ), supporting the notion that the inhibitory effect of LRP6N is via the direct interaction between LRP6 ectodomain and Frz. Importantly, CM containing the Wnt-unbinding LDLR had the same inhibitory effect ( Fig. 4d,e ). Among the LRP6 ectodomains, LDLR does not bind to Wnt ligands [8] , [9] , [10] , [11] ; therefore, these results further suggest the possibility that the inhibitory effect of LRP6N is not through binding to and neutralizing Wnt ligands but through the direct binding to Frz. LRP5/6 inhibit Frz function at the endogenous levels Wnt5a has been reported to activate the non-canonical pathway and induce migration of human melanoma cell line A2058 (ref. 16 ). We further used Wnt5a to examine the inhibitory role of LRP5/6 in endogenous Frz in A2058 cells. Consistent with the previous study, treatment with Wnt5a did promote A2058 cell migration, which was inhibited by pretreatment with LRP6N ( Fig. 5a,b ), supporting the notion that the inhibitory effect of LRP6 ectodomain is through direct binding to Frz. Knockdown of LRP5/6 but not β-catenin promoted migration of A2058 cells and the LRP5/6 knockdown-induced cell migration was greatly enhanced in response to Wnt5a treatment ( Fig. 5c ). These results indicate that endogenous LRP5/6 inhibit the Frz-regulated non-canonical pathway, and, therefore, in the absence of LRP5/6, A2058 cells have an enhanced response to Wnt5a. Of note, the inhibitory effect of endogenous LRP5/6 is canonical Wnt/β-catenin pathway-independent. 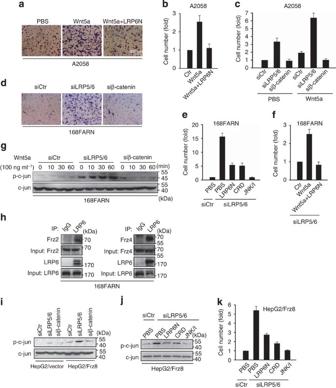Figure 5: LRP5/6 prevent Frz-mediated non-canonical pathway activation at the basal level. (a–f,k) Photoimages of transwell analysis and cell counting. In A2058 cells, Wnt5a promoted cell migration, which was completely inhibited by LRP6N (a,b). siRNA knockdown of LRP5/6 but not β-catenin promoted cell migration and the LRP5/6 knockdown-induced migration was further enhanced by treatment with Wnt5a (c). In 168FARN cells, siRNA knockdown of LRP5/6 but not β-catenin promoted cell migration (d). LRP5/6 knockdown-induced migration was impeded by LRP6N, CRD or JNK/I pretreatment in the upper chamber for 2 h (e), but further enhanced by treatment with Wnt5a (f). In HepG2/Frz8 cells, siRNA knockdown of LRP5/6 promoted cell migration (k). Scale bar, 300 μm. Values represent mean±s.d. of three experiments. (g,i,j) WB analysis of p-c-jun. siRNA knockdown of LRP5/6 (siLRP5/6) but not β-catenin increased the level of p-c-jun, which was enhanced by treatment with Wnt5a (100 ng ml−1) in 168FARN (g), and inhibited by LRP6N, CRD or JNK/I in HepG2/Frz8 cells (i,j);n=3. (h) IP/WB analysis showed the interaction between endogenous LRP6 and Frz2 (left panel) or Frz4 (right panel) in 168FARN cells;n=3. Figure 5: LRP5/6 prevent Frz-mediated non-canonical pathway activation at the basal level. ( a – f , k ) Photoimages of transwell analysis and cell counting. In A2058 cells, Wnt5a promoted cell migration, which was completely inhibited by LRP6N ( a , b ). siRNA knockdown of LRP5/6 but not β-catenin promoted cell migration and the LRP5/6 knockdown-induced migration was further enhanced by treatment with Wnt5a ( c ). In 168FARN cells, siRNA knockdown of LRP5/6 but not β-catenin promoted cell migration ( d ). LRP5/6 knockdown-induced migration was impeded by LRP6N, CRD or JNK/I pretreatment in the upper chamber for 2 h ( e ), but further enhanced by treatment with Wnt5a ( f ). In HepG2/Frz8 cells, siRNA knockdown of LRP5/6 promoted cell migration ( k ). Scale bar, 300 μm. Values represent mean±s.d. of three experiments. ( g , i , j ) WB analysis of p-c-jun. siRNA knockdown of LRP5/6 (siLRP5/6) but not β-catenin increased the level of p-c-jun, which was enhanced by treatment with Wnt5a (100 ng ml −1 ) in 168FARN ( g ), and inhibited by LRP6N, CRD or JNK/I in HepG2/Frz8 cells ( i , j ); n =3. ( h ) IP/WB analysis showed the interaction between endogenous LRP6 and Frz2 (left panel) or Frz4 (right panel) in 168FARN cells; n =3. Full size image We also found an inhibitory effect of endogenous LRP5/6 on the Frz-mediated non-canonical pathway in mouse breast tumour 168FARN cells. siRNA knockdown of LRP5/6 but not β-catenin in 168FARN cells induced cell migration ( Fig. 5d ). LRP5/6 knockdown-induced cell migration was inhibited by Frz8-CRD and JNK inhibitor ( Fig. 5e ) but enhanced by the treatment with Wnt5a ( Fig. 5f ), suggesting that endogenous LRP5/6 can prevent the activation of endogenous Frz-mediated non-canonical pathway. LRP5/6 knockdown-induced cell migration was also inhibited by LRP6N ( Fig. 5e,f ), suggesting that the ectodomain of LRP6 at the basal level prevents non-canonical pathway-mediated migration of mouse breast tumour cells. Furthermore, knockdown of LRP5/6 directly activated the non-canonical pathway downstream target c-jun, which was further enhanced by the treatment with Wnt5a ( Fig. 5g ). Notably, under basal condition or following β-catenin knockdown, 168FARN cells only had a weak response to Wnt5a ( Fig. 5g ). In attempting to determine the endogenous interactions between LRP5/6 and Frz using IP/WB analysis, we found that LRP6 bound to Frz2 and Frz4 in 168FARN cells ( Fig. 5h ), suggesting that endogenous LRP5/6 inhibit Frz through the direct LRP5/6–Frz interaction. RT-PCR assay showed that at least five Frzs including Frz2, Frz3, Frz4, Frz7 and Frz9 were expressed in 168FARN cells ( Supplementary Fig. 3 ). Whether LRP5/6 also interact with other Frzs in 168FARN cells warrants further investigation. Moreover, siRNA knockdown of LRP5/6 but not β-catenin in HepG2/Frz8 cells also increased the levels of phospho-c-jun ( Fig. 5i ). LRP5/6 knockdown-induced increase in the level of phospho-c-jun and cell migration was inhibited by LRP6N, Frz8-CRD and the JNK inhibitor ( Fig. 5j,k ). siRNA knockdown of β-catenin did not significantly change cell migration. As siRNAs of LRP5/6 and β-catenin in both mouse and human cells have the same effect, the off-target effects can be ruled out. In addition, LRP5/6 and β-catenin were shown to be effectively knocked down ( Supplementary Figs 4–6 ). Of note, 168FARN cells have almost undetectable expression levels of β-catenin ( Supplementary Fig. 7a ). Therefore, β-catenin is not actively involved in cell function, and the main function of LRP5/6 in 168FARN cells should be inhibiting non-canonical signalling through binding Frz, without interference from canonical Wnt/β-catenin signalling. As a result, knockdown of LRP5/6 in 168FARN cells induced a more marked cell migration pattern ( Fig. 5d,e ) than in A2058 cells ( Fig. 5c ) and HepG2/Frz8 cells ( Fig. 5k ). Taken together, these results indicate that the inhibitory effect of endogenous LRP5/6 on Frz is at least partially via the direct binding to Frz and is not related to the β-catenin-dependent canonical signalling pathway. LRP6 ectodomain prevents Frz-mediated metastasis in vivo 168FARN (non-metastatic) and 4T1 (metastatic) cells are subpopulations derived from the same mouse mammary tumour [27] . siRNA knockdown of endogenous LRP5/6 but not β-catenin in metastatic 4T1 cells marginally but significantly increased the levels of phospho-c-jun that was inhibited by LRP6N and Frz8-CRD ( Supplementary Fig. 8 ), as well as migration of 4T1 cells. The inhibitory effect of endogenous LRP5/6 in 4T1 cells was limited compared with that of 168FARN and A2058 cells, suggesting a cell context-dependency. However, treatment with LRP6N significantly decreased the level of phospho-c-jun and cell migration in 4T1 cells under basal condition ( Fig. 6a,b ). We next examined the role of LRP6N in preventing tumour metastasis using 4T1 cells in vivo . 4T1 cells implanted into the mammary fat pad formed macroscopic lung metastases, but 168FARN cells did not. At day 35 after implantation, representative micro-CT imaging and H&E staining of lungs showed anti-metastatic properties of LRP6N ( Fig. 6c,d ). As LRP6-unbinding Wnt5a was also able to promote migration of 4T1 cells, which was attenuated by pretreatment with LRP6N, suggesting that LRP6 ectodomain can prevent tumour cell metastasis in vivo at least partially by direct binding to Frz. 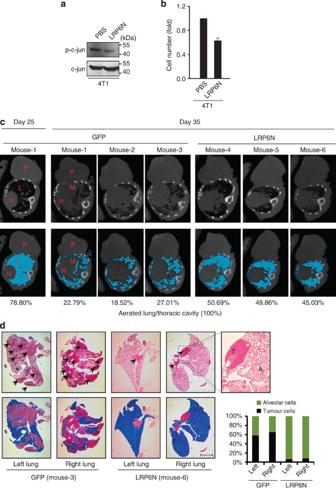Figure 6: LRP6 ectodomain prevents non-canonical pathway-regulated metastasis of mouse breast tumourin vivo. (a,b) WB analysis of p-c-jun and cell migration in cultured 4T1 cells. LRP6N attenuated c-jun activity (a) (n=3) and cell migration (b) at the basal level. Values represent mean±s.d. of three experiments. (c) Micro-CT images of the lungs were obtained from mice injected with LRP6N- or GFP-overexpressing 4T1 cells on day 25 and day 35. The multifocal tumour progression is clearly depicted from day 25 to day 35 in GFP-overexpressing mouse-1 and between LRP6N- and GFP-overexpressing mice at day 35. Axial slice orientation in corresponding positions. Segmentation of aerated lung (blue) was used as a surrogate parameter to assess the multifocal tumour spread (lower panels). The rate of aerated lung/thoracic cavity was higher in tumours from LRP6N-overexpressing 4T1 cells (∼48.53%) than GFP-overexpressing cells (∼22.77%), indicating less metastases in LRP6N-treated tumours. P=primary tumour; M=metastases; L=lung; H=heart. (d) Histology at day 35 showed distinctive tumour burden in corresponding areas by H&E staining. Arrow showed metastatic tumours. T=tumour cells; A=lung alveolar cells. Much more alveolar cells were present in LRP6N-overexpressing 4T1 cells than GFP-overexpressing cells (lower panel. blue colour and bar graph), indicating less metastases in LRP6N-treated tumours. Scale bar, 2 mm. Figure 6: LRP6 ectodomain prevents non-canonical pathway-regulated metastasis of mouse breast tumour in vivo . ( a , b ) WB analysis of p-c-jun and cell migration in cultured 4T1 cells. LRP6N attenuated c-jun activity ( a ) ( n =3) and cell migration ( b ) at the basal level. Values represent mean±s.d. of three experiments. ( c ) Micro-CT images of the lungs were obtained from mice injected with LRP6N- or GFP-overexpressing 4T1 cells on day 25 and day 35. The multifocal tumour progression is clearly depicted from day 25 to day 35 in GFP-overexpressing mouse-1 and between LRP6N- and GFP-overexpressing mice at day 35. Axial slice orientation in corresponding positions. Segmentation of aerated lung (blue) was used as a surrogate parameter to assess the multifocal tumour spread (lower panels). The rate of aerated lung/thoracic cavity was higher in tumours from LRP6N-overexpressing 4T1 cells ( ∼ 48.53%) than GFP-overexpressing cells ( ∼ 22.77%), indicating less metastases in LRP6N-treated tumours. P=primary tumour; M=metastases; L=lung; H=heart. ( d ) Histology at day 35 showed distinctive tumour burden in corresponding areas by H&E staining. Arrow showed metastatic tumours. T=tumour cells; A=lung alveolar cells. Much more alveolar cells were present in LRP6N-overexpressing 4T1 cells than GFP-overexpressing cells (lower panel. blue colour and bar graph), indicating less metastases in LRP6N-treated tumours. Scale bar, 2 mm. Full size image Of note, it is well known that the canonical pathway exerts potentially profound influence on tumour cell proliferation and survival, and plays a critical role in primary tumorigenesis [1] , [28] , [29] , [30] , [31] , [32] , [33] . LRP5/6 mutant lacking the cytoplasmic tail has been well established to inhibit canonical Wnt/β-catenin signalling through binding to and neutralizing Wnt ligands as described above [19] , [22] , [23] , [24] . Thus, to exclude the possibility that LRP6N prevents cell migration through inhibiting canonical Wnt/β-catenin signalling, we examined the level of nuclear β-catenin in HepG2/Frz8 cells and 4T1 cells following treatment with LRP6N. Indeed, we found nuclear β-catenin was not downregulated in HepG2/Frz8 cells by administration of soluble LRP6N ( Supplementary Fig. 9a ), as well as in 4T1 cells both in vitro and in vivo by transfection with plasmid carrying LRP6N ( Supplementary Fig. 10a,c ). In addition, LRP6N had no effect on cell proliferation in these two cells in vitro ( Supplementary Fig. 9b and 10b ) and tumour growth in vivo ( Supplementary Fig. 10d ). Thus, because LRP6N inhibits Wnt/β-catenin signalling through binding to and neutralizing Wnt ligands and that LRP6N did not decrease the levels of nuclear β-catenin in these two cells, these results suggest that the secretion of Wnt ligands in these cells is lacking. To further verify this notion, we examined β-catenin activity using a TOPFLASH assay. LRP6N had no effect on TOPFLASH activation at the basal levels in these two cells as well as in HEK293 cells; however, LRP6N inhibited TOPFLASH activation induced by transfection with canonical Wnt ligand Wnt3a in these cells ( Supplementary Fig. 1a–c ). As transfected Wnt3a should have much higher expression level than endogenous Wnt ligands, these findings suggest that these cells do in fact lack the secretion of Wnt ligands at the basal levels. In combination with the findings that LRP6N could inhibit the activation of non-canonical downstream target c-jun ( Figs 4a and 6a ), we can thus rule out the possibility that the inhibitory effects of LRP6N on cell migration are due to the inhibition of canonical Wnt/β-catenin signalling. Furthermore, β-catenin knockdown by siRNA in 168FARN cells and A2058 cells ( Fig. 5c,d ) as well as in 4T1 cells and HepG2/Frz8 cells did not induce cell migration, providing direct evidence that canonical Wnt/β-catenin signalling is not involved in cell migration, at least under our experimental conditions. Therefore, the inhibitory effects of LRP6N on HepG2/Frz8 cell migration ( Fig. 4 ) and 4T1 tumour metastasis in vivo ( Fig. 6 ) could be mainly due to its inhibition of non-canonical signalling pathway. Downregulation of membrane LRP5/6 in metastases LRP5/6 are presently thought to be required for mammary outgrowths and often overexpressed in breast tumours [4] , [5] , [6] , [7] . Higher expressions of LRP5/6 were also observed in metastatic 4T1 cells than non-metastatic 168FARN cells ( Supplementary Fig. 7b ). However, our present experiments show that downregulation of LRP5/6 seem crucial for tumour metastasis, thus it is noteworthy to observe the changing pattern of LRP5/6 expression during the course of breast cancer progression. As endogenous LRP5/6 are able to impede non-canonical pathway activation induced by the recombinant Wnt5a protein applied to cultured A2058 and 168FARN, LRP5/6 are supposed to impede the Frz-regulated non-canonical pathway mainly on the cell membrane. We thus compared the membrane expression level of LRP5/6 between primary tumour and metastases. Either or both of LRP5 and LRP6 were downregulated in lung metastases in all four 4T1 cell-xenografted mice ( Fig. 7a ). These data raise the possibility that downregulation of LRP5/6 is critical for mouse breast cancer metastasis. We also extended our analyses by determining LRP5/6 expression in tumour samples collected from 26 breast cancer patients. Both LRP5 and LRP6 were downregulated in lymph node metastases in 18 of the 26 patients ( Fig. 7b ). LRP5 was downregulated but LRP6 had similar expression in 2 out of 26 patients ( Fig. 7c ), whereas LRP6 was downregulated but LRP5 had similar expression in 4 out of 26 patients ( Fig. 7c ). In contrast, only 2 out of 26 patients showed higher expression levels of both LRP5 and LRP6 in lymph node metastases ( Fig. 7d ). Thus, 92.3% of patients showed downregulated expression of LRP5 or LRP6 in metastases, whereas only 7.7% of patients showed higher expression levels of LRP5 and LRP6 in lymph node metastases. Of note, low basal expression levels of both LRP5 and LRP6 (such as sample 22, 24, and 25) were observed in some patients, suggesting a limited ability of LRP5/6 in inhibiting the non-canonical pathway in these patients. Taken together, these in vivo experimental and clinical data suggest that downregulation of membrane LRP5/6 is crucial for tumour metastasis. 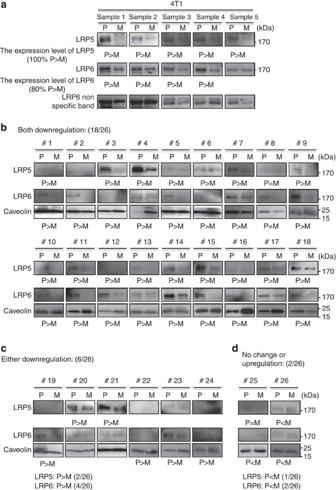Figure 7: Downregulation of membrane LRP5/6 in metastases of mouse and human breast tumours. (a–d) WB analysis showed lower level of membrane fraction in either or both of LRP5 and LRP6 in all lung metastases than in implanted primary 4T1 cells (a) in 92.3% of all patient lymph node metastases than in primary breast tumours (b–d). P=primary tumour; M=metastases. Figure 7: Downregulation of membrane LRP5/6 in metastases of mouse and human breast tumours. ( a – d ) WB analysis showed lower level of membrane fraction in either or both of LRP5 and LRP6 in all lung metastases than in implanted primary 4T1 cells ( a ) in 92.3% of all patient lymph node metastases than in primary breast tumours ( b – d ). P=primary tumour; M=metastases. Full size image Our present findings reveal a novel inhibitory mechanism of non-canonical Wnt signalling pathway by the direct interaction between LRP5/6 and Frz. According to our present observations, we propose a working model, in which, the LRP5/6–Frz complex maintains both canonical and non-canonical pathways in an inactive status at the basal level ( Fig. 8c ). However, to transduce signals, canonical Wnt ligand like Wnt1 or Wnt3a induce a conformational change of the LRP5/6-Frz complex but does not significantly change the relative positions of LRP5/6 and Frz ( Fig. 8b ). In contrast, non-canonical Wnt ligand Wnt5a strongly activates the non-canonical pathway in the absence of LRP5/6 ( Fig. 8d ), but weakly activates the pathway in the presence of LRP5/6 ( Fig. 8e ). 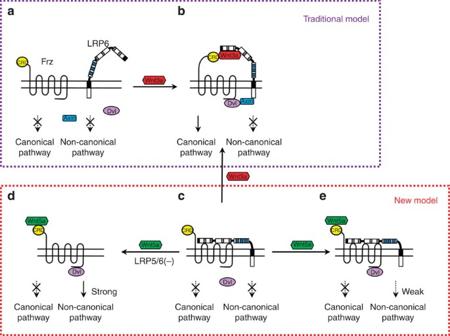Figure 8: A novel working model of the canonical and non-canonical pathways. (a–e) Schematic illustration of the role of LRP5/6 in regulating canonical and non-canonical Wnt signal transduction. The traditional model (a,b). LRP5/6 and Frz form a complex at the basal state, and this ligand-independent interaction maintains the receptor complex in an inactive state (c). Non-canonical Wnt ligand Wnt5a strongly activates the non-canonical pathway in the absence of LRP5/6 (d), but weakly activates the pathway in the presence of LRP5/6 (e). Figure 8: A novel working model of the canonical and non-canonical pathways. ( a – e ) Schematic illustration of the role of LRP5/6 in regulating canonical and non-canonical Wnt signal transduction. The traditional model ( a , b ). LRP5/6 and Frz form a complex at the basal state, and this ligand-independent interaction maintains the receptor complex in an inactive state ( c ). Non-canonical Wnt ligand Wnt5a strongly activates the non-canonical pathway in the absence of LRP5/6 ( d ), but weakly activates the pathway in the presence of LRP5/6 ( e ). Full size image It was previously shown that LRP6–Frz8 interaction is ligand-dependent [2] ; however, this conclusion was obtained from experiments using LRP6N and Frz8-CRD, and is not inconsistent with our observation that ligand-independent LRP6–Frz8 interaction is mediated by Frz8 beyond Frz8-CRD. As deregulation of Wnt signalling has been linked to various human diseases [1] , [2] , [9] , [15] , the mutual inhibition of LRP5/6 and Frz by this LRP5/6–Frz interaction at the basal level is crucial for maintenance of tissue homeostasis. In addition, the presence of LRP5/6 and Frz in the same complex is time-saving for locally secreted Wnt ligand to rapidly detect them and transduce signals. It has been reported that the combination of Wnt ligands, LRP6 and ATF3 had a significant inverse correlation with metastasis-free survival of prostate cancer patients [34] . Liu et al . showed that the tumour metastasis suppressor gene, NDRG1, prevented metastasis in prostate and breast cancer through inhibiting the canonical Wnt/β-catenin pathway. They first showed a physical interaction of NDRG1 with LRP6 and an inhibitory role of NDRG1 on LRP6. They then showed a higher expression of LRP6 mRNA in prostate metastatic tumour (of note, they compared the difference of LRP6 expression between different patients) and drew the conclusion that LRP6 expression had a significant inverse correlation with metastasis-free survival of prostate cancer patients. However, when they investigated how NDRG1 suppressed metastasis via suppressing the canonical pathway, they examined the role of β-catenin itself and the relationship between NDRG1 and β-catenin in regulating metastasis, but did not examine the role of LRP6. Therefore, the role of LRP6 in regulating metastasis remains unexplored in their study. Our present study presented several different points as summarized below: (1) we identified a β-catenin-independent role of LRP5/6 in inhibiting non-canonical pathway and cell migration; (2) we examined the role of not only LRP6 but also LRP5; (3) we compared the expressions of LRP5 and LRP6 between primary tumour and metastases in the same patient as well as in the same animal; (4) we compared their expressions in breast tumour rather than prostate tumour. We found that the expression levels of LRP5 and LRP6 were significantly downregulated in metastases compared with primary tumour in the same patient as well as in the same animal ( Fig. 7 ). In contrast, although our present findings show that downregulation of membrane LRP5/6 might be required for the initiation of both murine and human breast tumour metastasis, LRP6 is often overexpressed in human breast tumours [4] , [5] , [6] , [7] and higher expression of LRP5/6 is also observed in metastatic 4T1 cells compared with non-metastatic 168FARN cells ( Supplementary Fig. 7b ). An important point is that, if the canonical Wnt-LRP5/6-β-catenin pathway is important for metastasis, the expression levels of LRP5/LRP6 should be higher (or at least the same) in metastases than in primary tumours in the same cancer patient. However, our present study provided directly contrasting results, with lower expression levels of LRP5/LRP6 in metastases than in primary tumours both in human patients and murine experiments ( Fig. 7 ). Thus, although the high expressions of canonical pathway components such as LRP5/6 and β-catenin might be critical for cancer development, it is highly possible that the downregulation of LRP5/6 might also be critical for distant metastasis as shown in our present study. Therefore, upregulation of LRP5/6 is supposed to be initially critical for β-catenin-dependent tumorigenesis, but consequently downregulation from cell surface will eventually lead to β-catenin-independent non-canonical pathway-mediated tumour metastasis. Whether downregulation of membrane LRP5/6 also occurs in other tumour metastasis warrants further study. The mechanism by which membrane LRP5/6 are downregulated is still unclear. It is known that Wnt3a and Dkk1 can induce internalization of LRP5/6 (refs 35 , 36 ). Frz and LRP5/6 are internalized simultaneously in response to Wnt3a, but only LRP5/6 are removed from membrane in response to Dkk1 (refs 12 , 35 , 36 ). Thereby, Dkk1 might be the key factor for promoting tumour metastasis by downregulating membrane LRP5/6. Notably, cancer patients with Dkk1 upregulation have long been known to have poorer prognosis, although the reason remains unknown [37] . Our present findings also show a higher expression of Dkk1 in 4T1-implanted primary tumour than metastases, and no expression of Dkk1 was detected in neighbouring normal lung tissues ( Supplementary Fig. 11 ), suggesting a possibility that the removal of LRP5/6 from cell surface by Dkk1 upregulation relieves the inhibition of LRP5/6 on tumour metastasis regulated by Frz-induced non-canonical Wnt pathway activation. Indeed, our preliminary observation has shown that overexpression of Dkk1 promoted cell invasion in HepG2 cells ( Supplementary Fig. 12 ). Owing to the oncogenic role of canonical Wnt signalling [3] , [4] , [5] , [6] , [7] , [9] , [31] , [38] , upregulation of Dkk1 as a canonical pathway inhibitor might initially be beneficial for preventing canonical pathway-induced tumour growth. However, its persistent upregulation would downregulate membrane LRP5/6 and eventually induce non-canonical-regulated tumour metastasis. The dual actions of Dkk1 as a canonical inhibitor and non-canonical activator in cancer warrants further investigation. Increased autocrine canonical Wnt ligands and LRP5/6 receptors at the cell surface have been associated with tumour development and progression [3] , [4] , [7] , [39] . These previous observations have provided rationale for the development of anti-LRP6 antibodies aimed at inhibiting LRP6 function [40] , [41] . According to our present LRP5/6-Frz interaction model, the application of anti-LRP6 antibodies that block Wnt ligand-mediated β-catenin signalling requires possible reconsideration because competitive interaction of these antibodies might separate Frz from LRP6 to activate the Frz-regulated non-canonical pathway and result in tumour metastasis. Until recently, only a few metastasis suppressor genes had been characterized [42] . The ascertained downregulation of either or both of LRP5 and LRP6 in metastatic mouse and human breast cancer carries significant implications regarding our understanding of the pathogenesis of high-grade malignancies. The dual roles of LRP5/6 as oncogenes and metastasis suppressor genes would be promising therapeutic targets for cancer development and metastasis and as significant prognostic markers. Owing to the role of LRP6 ectodomain in binding and then neutralizing Dkk1 to prevent non-canonical pathway activation, as well as inhibiting both canonical and non-canonical pathways through binding to Frz and Wnt ligands, a rapid clinical advancement for cancer treatment by soluble LRP6N protein would be worthwhile. BRET assay BRET assays [21] were performed essentially as follows. 293T cells were transfected with various combinations of expression vectors for GFP2-tagged proteins, Rluc8-tagged proteins and Mesd. Twenty-four hours after transfection, cells were collected in OPTI-MEM (Invitrogen, USA) and replated in 96-well plates. BRET activities were measured 1 h after replating using a microplate reader LB940 (Mithras) with coelenterazine 400A (Biotium, USA) as a substrate at a final concentration of 5 mM. Light emissions were measured in 370–450 nm for Rluc8 and 495–535 nm for GFP2. Where indicated, Wnt3a was added at a concentration of 1,000 ng ml −1 . Primary tumour material The investigation complied with the principles that govern the use of human tissues outlined in the Declaration of Helsinki. We have obtained informed consent from all patients. The breast tumours and the distant metastases were obtained from The Department of Breast Surgery, The Affiliated Tumour Hospital, Guangxi Medical University, with appropriate ethical approval from the repositories. Western blot and IP/western blot analysis Conditioned media containing LRP6 deletion mutants were produced with HEK293 cells. Plasmids were transiently transfected into HEK293 cells and IP was performed with Protein G–Sepharose 4 Fast Flow (Amersham, USA). To examine the effect of Wnt ligand sequestration on Frz8-LRP6 interaction in HepG2 cells, an expression vector for Frz8-CRD-IgG/Fc was transfected 48 h before harvest. Membrane protein extraction kit was purchased from Beyotime Institute of Biotechnology (Beyotime, CHN). Tumour tissue or cells were lysed in RIPA (50 mM Tris (pH 7.4), 150 mM NaCl, 1% Triton X-100, 1% sodium deoxycholate, 0.1% SDS, sodium orthovanadate, sodium fluoride, EDTA and leupeptin) (Beyotime, CHN). The lysates were heated to 95 °C, separated by SDS–PAGE and transferred to PVDF membranes. The membranes were blocked with 5% skim milk for 1 h and incubated overnight at 4 °C with the appropriate primary antibodies. The antibodies used for IP and western blotting were from Invitrogen (anti-myc 1:1,000 and anti-V5 1:1,000), Sigma (anti-Flag 1:1,000), Santa Cruz (anti-LRP5 1:1,000, anti-LRP6 1:1,000 and anti-Frz8 1:1,000), Cell Signaling (anti-phospho-LRP6 1:1,000, anti-phospho-c-jun 1:1,000 and anti-c-jun 1:1,000) and Beyotime (anti-β-actin 1:1000). After incubation with horseradish peroxidase-conjugated secondary antibodies for 1 h at room temperature, the immunoblots were visualized using enhanced chemiluminescence (Pierce). Uncropped scanned images of western blots are presented in Supplementary Fig. 13 . FAR-WB analysis FAR-WB analysis was performed as previously described [20] . In brief, 48 h after transfection of V5-tagged Frz8 in HEK293 cells, cell lysates were separated by standard denatured SDS-–PAGE and transferred to PVDF membrane. After re-naturation of V5-Frz8 on PVDF membrane with gradient guanidine hydrochloride, the PVDF membrane was incubated with myc-tagged LRP6N protein (1 mg ml −1 ) purified by myc agarose affinity column, and the existence of the myc-LRP6N was detected at the expected position of Frz8. Reporter gene assay Luciferase activity was examined using Luciferase Assay kit (Promega, E1980). In brief, after transfection of TOPFLASH reporter gene together with LRP6 mutants or Frz8 mutants using Fugene (Roche) in 48–well plate (3 × 10 4 cells per well) for 48 h, lysates of HEK293 cells were measured according to the assay kit protocol. All data were normalized by Renilla activity. Transwell assay Cells were seeded on 35-mm dishes and were transfected using RNAiMAX (Invitrogen, USA). After 48 h, the cells (4 × 10 5 cells) in serum-free culture medium were seeded into the upper chamber of Transwell 24-well plates (8 μm polycarbonate membrane (Corning, USA)). The inhibitors (LRP6N-IgG/Fc, Frz8-CRD-IgG/Fc and JNK inhibitor) were added into the upper chamber. After 24 h, cells that migrated through the filter into the bottom chamber were stained by Toluidine Blue O (Sigma) and counted. The number of migrating cells was normalized to control conditions and expressed as a migration index. Animal model All animal protocols were approved by the Animal Care and Use Committee at the Tongji University School of Medicine and followed the NIH Guidelines for Care and Use of Animals in Research (NIH Publication No. 85-23, revised 1996). Severe combined immune deficiency mice were used for the mammary orthotopic implant. A plasmid with LRP6N or GFP was transfected into 4T1 cells using the polysaccharide-based Dextran-g-PEIs method [43] , and, after 48 h, 5 × 10 5 cells were injected into mice under the mammary fat pad. Seven days after implantation, the plasmid was injected into the primary tumour again using the polysaccharide-based Dextran-g-PEIs method [43] . Tumours in the lungs were identified via micro-CT imaging and histology examination. For histology examination, the left and right lungs of each animal were fixed in 4% formalin and sections were stained with haematoxylin and eosin (H&E). Micro-CT Non contrast-enhanced prospectively respiratory-gated micro-CT was performed (Triumph-XO-CT Pre-Clinical Imaging System, Gamma Medica-Ideas, US) with an effective pixel size of 0.05 mm (75 kV, 150 μA, 512 projections/scan, exposure time/projection 250 ms, ‘fly’ data acquisition mode, 2 × 2 detector bin mode, 0.1 mm thickness/projection). The scan FOV was 35.84 mm. Images of the chest were reconstructed and calibrated to the Hounsfield scale. A Gaussian filter was used to reduce noise in the grey-scale images. All images were viewed in lung window and soft tissue window by GEHC Microview2.4. Plasmids and reagents TOPFLASH reporter was from RT. Moon [32] , [44] . Full-length Frz8, Frz8-CRD-IgG/Fc and LRP6N expression vectors were from X. He [19] , [45] . Full-length LRP6, membrane-bound forms of LRP6 deletion mutants, Dkk1, and Kremen2 were from C. Niehrs [11] , [12] . Frz3 and Frz4 were from Nathans, J [46] . Rluc8 was from SS. Gambhir [47] . GFP2 was purchased from Perkin Elmer. Mesd was from BC. Holdener [48] . Other LRP6 mutants were generated with a QuickChange Site-Directed Mutagenesis kit (Stratagene, USA). Wnt5a, Dkk1, LRP6N-IgG/Fc and Frz8-CRD-IgG/Fc were purchased from R&D, USA. Human and mouse siRNAs, and transfection reagent RNAiMAX were purchased from Invitrogen, USA. Transfection reagent Fugene was from Roche, Switzerland. Statistics All data are expressed as the mean±s.e.m. In all experiments, an unpaired t -test with Welch’s correction or a one-way analysis of variance was used to compare experimental groups with their appropriate control unless otherwise specified; P <0.05 was considered significant for all experiments. How to cite this article: Ren, D.-n. et al . LRP5/6 directly bind to Frizzled and prevent Frizzled-regulated tumour metastasis. Nat. Commun. 6:6906 doi: 10.1038/ncomms7906 (2015).